Unusually stable ~100-fold reversible and instantaneous swelling of inorganic layered materials Cells can swell or shrink in certain solutions; however, no equivalent activity has been observed in inorganic materials. Although lamellar materials exhibit increased volume with increase in the lamellar period, the interlamellar expansion is usually limited to a few nanometres, with a simultaneous partial or complete exfoliation into individual atomic layers. Here we demonstrate a large monolithic crystalline swelling of layered materials. The gallery spacing can be instantly increased ~100-fold in one direction to ~90 nm, with the neighbouring layers separated primarily by H 2 O. The layers remain strongly held without peeling or translational shifts, maintaining a nearly perfect three-dimensional lattice structure of >3,000 layers. First-principle calculations yield a long-range directional structuring of the H 2 O molecules that may help to stabilize the highly swollen structure. The crystals can also instantaneously shrink back to their original sizes. These findings provide a benchmark for understanding the exfoliating layered materials. Two-dimensional (2D) atomic crystals or nanosheets—individual atomic planes peeled from bulk-layered materials—have emerged as an important family of nanoscale materials because of their fascinating properties and diverse applications [1] , [2] , [3] . Inorganic materials with layered structures that serve as precursors for 2D nanosheets contain loosely stacked host layers that display layer-to-layer gallery expansion or swelling upon the intercalation of certain ions and/or solvents [4] , [5] , [6] , [7] , [8] . The swelling, however, is generally limited, with lamellar periods larger than a few nanometers only occurring in rare cases. Exfoliation, in which the layered phase is cleaved into nanosheets, typically accompanies the swelling due to the rapidly weakened electrostatic attractions between the layers [6] , [8] , [9] , which produce colloidal dispersions of the individual 2D layers or sheets. For example, graphite oxide, also called ‘graphitic acid’, demonstrates some degree of swelling through hydration when immersed in pure or basic water, with its layers easily separated, producing colloidal suspensions of graphene oxide [10] . Despite continuous efforts to exfoliate various layered materials, including graphite, [11] boron nitride, [12] , [13] layered metal chalcogenides, [1] oxides, [3] , [14] , [15] , [16] and hydroxides, [3] , [17] studying a highly swollen structure, which is required to understand the exfoliation process and 2D crystals, remains a great challenge given the low structural stability of the swollen phases. We demonstrate a reversible swelling and shrinkage of up to ~100-fold, with a maximum periodicity of ~90 nm, induced by polar amines. Despite the large interlayer distances, the >3,000 atomic layers exhibit no signs of breakage or exfoliation into individual sheets and move apart and instantly return together in a manner similar to springing poker cards. The driving force that initiates the insertion of an ion and/or water into the galleries is an acid–base reaction, and the process is precisely controlled by the acid–base equilibrium and osmotic pressure equilibrium between the gallery inside and solution reservoir outside. A variety of protonated oxides or solid acids manifest such behaviours, such as H 1.07 Ti 1.73 O 4 ·H 2 O, H 2 Cs 4 W 11 O 36 ·6H 2 O, HCa 2 Nb 3 O 10 ·1.5H 2 O, and so on. This study examines H 0.8 [Ti 1.2 Fe 0.8 ]O 4 ·H 2 O, a typical layered material, as an example. The unusual high stability of the newly developed swollen structure was interpreted using a first-principle study to demonstrate the formation of ordered H 2 O dipoles between the layers, unlike the previously reported random H 2 O molecules in normal swollen phases that are easily exfoliated. The stability of the swollen phases is largely determined by the chemical nature of the ions that enter into the gallery and their interactions with the surrounding H 2 O molecules. Characterization of the swollen crystals We chose H 0.8 [Ti 1.2 Fe 0.8 ]O 4 ·H 2 O for a representative study because the crystals are of suitable size for observing the swelling process in situ using an optical microscope (see Supplementary Fig. S1 for the swelling of other crystals). Single crystals of H 0.8 [Ti 1.2 Fe 0.8 ]O 4 ·H 2 O with lateral sizes of ~15 μm × 35 μm and a thickness of ~2–3 μm were obtained through proton-exchange reactions with the parent compound K 0.8 [Ti 1.2 Fe 0.8 ]O 4 ( Fig. 1a ), which was prepared using a flux method. Previous studies have reported that H 0.8 [Ti 1.2 Fe 0.8 ]O 4 ·H 2 O crystallizes in an orthorhombic structure containing negatively charged layers [Ti 0.6 Fe 0.4 ]O 2 0.4− stacked along the [010] direction, with charge-balancing ions and water molecules in the gallery ( Fig. 2c ) [14] . The gallery spacing is 0.89 nm; thus, the platelets are composed of ~3,000 regularly stacked layers. 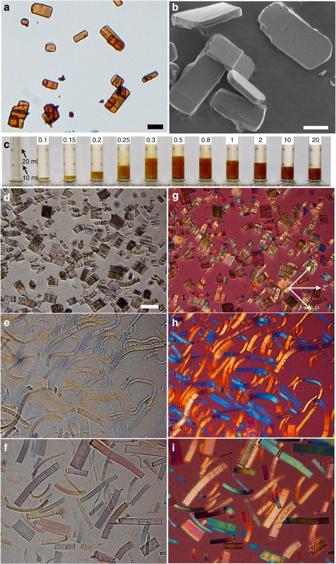Figure 1: Macroscopic volume and microscopy characterization of the samples before and after swelling. (a) Optical microscopy and (b) scanning electron microscopy images of the parent K0.8[Ti1.2Fe0.8]O4microcrystals exhibiting platelets with lateral sizes of ~15 μm × 35 μm and a thickness of ~2–3 μm. The scale bars inaandbrepresent 20 μm and 10 μm, respectively. (c) Photograph showing the changes in macroscopic volume of the swollen crystals in 100 ml of various DMAE solutions. The yellow-brown swollen phases settle at the bottom of the graduated cylinders. The leftmost sample is the original H0.8[Ti1.2Fe0.8]O4·H2O microcrystal sample before swelling, which is presented for comparison. (d–f) Optical microscopy images showing the extended lamellar structures of the typical swollen phases at DMAE/H+=0.1, 0.5 and 10. Observations were made by dropping one or two drops of the swollen samples, shown inFig. 1c, onto glass slides. The longest swollen length is ~200–250 μm in DMAE/H+=0.5. At high concentrations, the swelling is somewhat suppressed, with swollen length of ~100 μm at DMAE/H+=10. (g–i), The swollen samples observed via crossed polarizers. The images were collected with a 530 nm sensitive colour plate inserted into the light path. InFig. 1g, P and A represent the axes of the polarizer and analyzer, respectively. Z′ represents the slow axis of the sensitive colour plate. Iridescence was typically observed in crystallites swollen in DMAE/H+=0.1, suggesting a heterogeneous nature. Other samples reveal homogeneous swelling, with no change in the interference colour within a crystallite. All optical microscopy images were obtained at the same magnification. Scale bar, 50 μm. Figure 1: Macroscopic volume and microscopy characterization of the samples before and after swelling. ( a ) Optical microscopy and ( b ) scanning electron microscopy images of the parent K 0.8 [Ti 1.2 Fe 0.8 ]O 4 microcrystals exhibiting platelets with lateral sizes of ~15 μm × 35 μm and a thickness of ~2–3 μm. The scale bars in a and b represent 20 μm and 10 μm, respectively. ( c ) Photograph showing the changes in macroscopic volume of the swollen crystals in 100 ml of various DMAE solutions. The yellow-brown swollen phases settle at the bottom of the graduated cylinders. The leftmost sample is the original H 0.8 [Ti 1.2 Fe 0.8 ]O 4 ·H 2 O microcrystal sample before swelling, which is presented for comparison. ( d – f ) Optical microscopy images showing the extended lamellar structures of the typical swollen phases at DMAE/H + =0.1, 0.5 and 10. Observations were made by dropping one or two drops of the swollen samples, shown in Fig. 1c , onto glass slides. The longest swollen length is ~200–250 μm in DMAE/H + =0.5. At high concentrations, the swelling is somewhat suppressed, with swollen length of ~100 μm at DMAE/H + =10. ( g – i ), The swollen samples observed via crossed polarizers. The images were collected with a 530 nm sensitive colour plate inserted into the light path. In Fig. 1g , P and A represent the axes of the polarizer and analyzer, respectively. Z′ represents the slow axis of the sensitive colour plate. Iridescence was typically observed in crystallites swollen in DMAE/H + =0.1, suggesting a heterogeneous nature. Other samples reveal homogeneous swelling, with no change in the interference colour within a crystallite. All optical microscopy images were obtained at the same magnification. Scale bar, 50 μm. 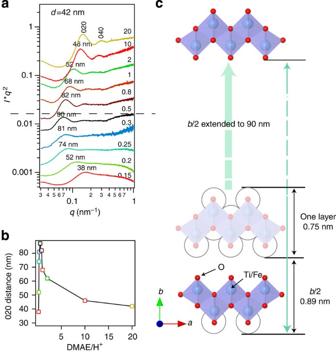Figure 2: Evidence of crystalline swelling using SAXS. (a) SAXS profiles of the typical samples collected on the beamline BL11 at the Kyushu Synchrotron Light Research Center using a fixed wavelength of 0.177 nm. Several drops of the swollen crystals that settled at the bottom of graduated cylinders, as shown inFig. 1c, were packed into a 2 mm-deep sample cell that was sealed with a Kapton film to prevent solvent evaporation during the measurements. The products of the scattering intensity,I, and the inverse of form factor of a flat, thin sheet (q2),I*q2, were plotted against the scattering vector modulus,q. The correspondingd-spacing values were calculated using the formulad=2π/q. (b) Evolution of the lamellar period,d, with DMAE/H+. (c) An illustration of the swollen structure. Compared with the crystal structure of the original H0.8[Ti1.2Fe0.8]O4·H2O, which is composed of [Ti0.6Fe0.4]O20.4−layers stacked with a spacing of 0.89 nm, the interlayer distance increased to 90 nm, resulting in ~100-fold swelling. Full size image Figure 2: Evidence of crystalline swelling using SAXS. ( a ) SAXS profiles of the typical samples collected on the beamline BL11 at the Kyushu Synchrotron Light Research Center using a fixed wavelength of 0.177 nm. Several drops of the swollen crystals that settled at the bottom of graduated cylinders, as shown in Fig. 1c , were packed into a 2 mm-deep sample cell that was sealed with a Kapton film to prevent solvent evaporation during the measurements. The products of the scattering intensity, I , and the inverse of form factor of a flat, thin sheet ( q 2 ), I * q 2 , were plotted against the scattering vector modulus, q . The corresponding d -spacing values were calculated using the formula d =2 π / q . ( b ) Evolution of the lamellar period, d , with DMAE/H + . ( c ) An illustration of the swollen structure. Compared with the crystal structure of the original H 0.8 [Ti 1.2 Fe 0.8 ]O 4 ·H 2 O, which is composed of [Ti 0.6 Fe 0.4 ]O 2 0.4− layers stacked with a spacing of 0.89 nm, the interlayer distance increased to 90 nm, resulting in ~100-fold swelling. Full size image To induce swelling, the crystals were exposed to aqueous amine solutions. In this report, 2-(dimethylamino)ethanol (DMAE, (CH 3 ) 2 NC 2 H 4 OH) will be addressed in detail (see Supplementary Fig. S2 for details regarding swelling with other amines, such as 3-dimethylamino-1-propanol, 4-amino-1-butanol, and so on). The samples ‘ballooned’ spontaneously and were kept still overnight to achieve equilibrium. The swelling was controlled by varying the DMAE concentration. The DMAE concentrations ranged from 0.00086 to 0.1702, mol/l, which corresponds with a 0.1- to 20-fold excess the ion-exchange capacity of the H 0.8 [Ti 1.2 Fe 0.8 ]O 4 ·H 2 O ( Fig. 1c ). The volume increased even in dilute DMAE solutions, including DMAE/H + =0.1 ( C DMAE =0.00086, mol/l), in which H + represents exchangeable protons in the solid (0.8 per formula weight of H 0.8 [Ti 1.2 Fe 0.8 ]O 4 ·H 2 O). The volume increased with increasing DMAE concentrations and reached a maximum at DMAE/H + =0.5; however, the volume decreased at higher concentrations. Optical microscopy characterization of the representative samples of DMAE/H + =0.1, 0.5 and 10 ( Fig. 1d–i ; for others, see Supplementary Fig. S3 ) revealed extended lamellar structures, with average lengths ranging from 50 μm to 250 μm, depending on the initial DMAE concentration. This finding corroborates the anisotropic swelling of the original crystals that occurs perpendicular to the plane of the host layers. Observations made with a crossed polarizer suggest that the swelling is homogeneous and exhibits no change in the interference colour along a crystallite edge, except with the DMAE/H + =0.1 sample. Some crystallites in the DMAE/H + =0.1 sample appear to be in the intermediate stage of swelling and exhibit iridescent colours ( Fig. 1g ), suggesting that heterogeneous swelling occurs at low concentrations. The average swollen length, ~200–250 μm ( Fig. 1e ), was longest for the samples swollen at DMAE/H + =0.5. Given an original crystal thickness of ~2–3 μm, crystal swelling up to ~100-fold is surprising. The repeat distances in the stacked sheets of the swollen samples were further examined using small-angle X-ray scattering (SAXS). Figure 2a shows the SAXS profiles of representative samples. A single diffuse peak at d =35 nm was barely detectable in samples swollen at DMAE/H + =0.1 ( Supplementary Fig. S4 ), which supports the heterogeneity observed with the microscope. The samples that swell at higher concentrations presented patterns with distinct maxima. The patterns evolved from one broad peak to the presence of double well-defined reflections, which can be assigned to the 020 and 040 basal reflections in the lamellar phase and confirm the unidimensional swelling. The reflection peaks simultaneously became better defined and stronger with increasing concentration, suggesting a decrease in the spacing fluctuations. The observed spacings ( Fig. 2b ) confirmed those obtained using the optical microscope, indicating that the crystals swell homogeneously as a monolithic body and do not cleave into thinner pieces. The crystals exhibited a maximum swelling in DMAE/H + =0.5, which produces a basal spacing, d , of 90 nm. Therefore, the lamellar swollen phase consisted of a repeated crystalline stack of titanate sheets that were 0.75 nm thick, with a controllable periodicity up to 90 nm ( Fig. 2c ). In dilute DMAE solutions (DMAE/H + <0.5), the d value of the swollen crystals increased almost linearly with increasing concentration, which revealed a progressive increase in the intake of water molecules. The interplanar spacing decreased rapidly to 68 nm for DMAE/H + =1 and leveled off in concentrated solutions, showing little variation (46 nm, 42 nm and 40 nm at DMAE/H + =10, 20 and 100, respectively). This changing trend could be qualitatively explained using a modified Derjaguin–Landau–Verwey–Overbeek theory or the Sogami-Ise theory, [9] with the parameters summarized in Supplementary Table S1 . The swollen spacings predicted at high concentrations correspond with the experimental values ( Supplementary Methods ; Supplementary Fig. S5 ). The highly swollen crystalline structure of regularly stacked atomic sheets demonstrated both long-range orientational and positional order, and possessed certain layer-to-layer interactions, which differed from those of the liquid crystalline nanosheets that form at high concentrations. [18] , [19] , [20] , [21] , [22] For example, a liquid crystalline lamellar phase was prepared from colloidal suspensions of H 3 Sb 3 P 2 O 14 sheets, [18] with a layer-to-layer distance that was 100-fold than that in the original crystal structure. Graphite spontaneously exfoliates into single-layer graphene and forms liquid crystalline phases at high concentrations. [22] The liquid crystal phase is an orientational ordering of the nanosheets driven by entropy loss that decreases the positional order and eliminates the sheet-to-sheet registry between neighboring nanosheets. Swelling and shrinking of the crystals observed in real time The stable ~100-fold increase in volume occurred rapidly in just a few seconds. We observed the swelling process in real time using an optical microscope following a one-drop addition of the DMAE solution ( Fig. 3 ). The real-time movie is provided in the Supplementary Movie 1 . The volume increase occurred immediately after the DMAE addition, and the crystals swelled beyond 200 μm in 1.4 s. However, little growth was observed after another 15 s. The swelling was reversible. Upon the addition of HCl, the water molecules were eliminated, and the crystals shrank back to their original sizes ( Fig. 3f–h ). In both processes, the crystal grew and shrank homogeneously as a unit without thinning or falling apart. 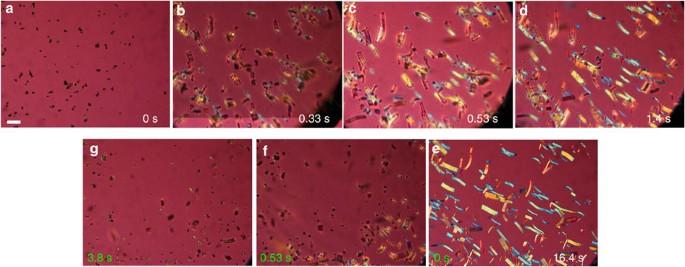Figure 3:Time-series images of the H0.8[Ti1.2Fe0.8]O4·H2O crystals. (a) Image of the starting materials. (b–e) Images collected at 0.33, 0.53, 1.4 and 16.4 s after the addition of one drop of the DMAE solution. (f,g) HCl was added, and the swollen crystals instantaneously shrank back to their original size. Scale bar, 100 μm. Figure 3: Time-series images of the H 0.8 [Ti 1.2 Fe 0.8 ]O 4 ·H 2 O crystals. ( a ) Image of the starting materials. ( b – e ) Images collected at 0.33, 0.53, 1.4 and 16.4 s after the addition of one drop of the DMAE solution. ( f , g ) HCl was added, and the swollen crystals instantaneously shrank back to their original size. Scale bar, 100 μm. Full size image Concentration difference between the gallery and surrounding reservoir The system can be simplified by being divided into two regions, swollen ‘aquacrystals’ and the surrounding solution reservoir, by an imaginary semipermeable membrane, as illustrated by the dotted line in Fig. 4a . This model is comparable to a cell suspended in a liquid. In aqueous solutions, the amine end of the DMAE tends to accept a proton from water because of the presence of lone electron pairs, generating [HN(CH 3 ) 2 C 2 H 4 OH] + (DMAEH + ), which can passively diffuse between the two regions along with the H + and OH – . However, the negatively charged host layers remain in the internal region. The swelling, or influx of DMAE solution, is thought to be initiated by acid–base reactions between the protons in the crystal gallery and DMAE, which is a weak base in aqueous media. Similar to that within a cell, the mobility of the various species is driven by osmotic pressure. Therefore, the swelling process is a delicate balance between an acid–base equilibrium and osmotic pressure equilibrium, the destruction of which may shrink the swollen samples as what occurs after HCl addition. 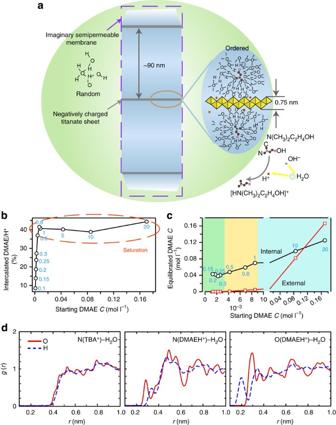Figure 4:Distribution of DMAE and H2O molecules. (a) Illustration of the system divided into two regions that are similar to a cell suspended in liquid. The broken line represents an imaginary semipermeable membrane at the boundary of the two regions. The negatively charged host layers remain only in the internal region, resulting in concentrated DMAEH+in the gallery as determined by the Gibbs–Donnan equilibrium. Unlike the bulk water in the external reservoir, the strong interactions between the DMAEH+and H2O trigger the formation of an orientated hydrogen-bonded network that could help to stabilize the lamellar structure and connect the successive layers separated by up to 90 nm. (b) The amount of intercalated DMAE molecules (as a percentage of the exchange capacity) provided as a function of the initial DMAE concentration. The amount of intercalated DMAE molecules first increased sharply in a nearly linear manner until reaching a saturation value at DMAE/H+= ~0.5–1, which is ~37% of the exchange capacity. This corresponded with the maximum swelling, beyond which no additional solvent could penetrate between the sheets. (c) A comparison of the DMAE concentrations inside and outside of the gallery. The DMAE typically concentrates in the gallery. Under the dilute regime before saturation, the external concentrations approached zero, while the internal concentrations remained nearly constant (0.04 mol l−1). The reverse occurred at high concentrations, beyond which little change in swelling was observed. (d) The radial distribution functionsg(r) of water from nitrogen in TBAOH and DMAE and from oxygen (–OH) in DMAE. The solid and broken lines denote the water oxygen and hydrogen, respectively. The water molecules surrounding DMAEH+exhibited substantially higher-ordered structures than the random state around the TBA+. Furthermore, the –NH and –OH in the DMAEH+attracted O and H, respectively, of the polar H2O, producing water clusters with a net dipole (Supplementary Fig. S8). The ‘polar’ water clusters interconnected through the dipole–dipole interactions, which may have helped to stabilize the highly swollen structure. Figure 4: Distribution of DMAE and H 2 O molecules. ( a ) Illustration of the system divided into two regions that are similar to a cell suspended in liquid. The broken line represents an imaginary semipermeable membrane at the boundary of the two regions. The negatively charged host layers remain only in the internal region, resulting in concentrated DMAEH + in the gallery as determined by the Gibbs–Donnan equilibrium. Unlike the bulk water in the external reservoir, the strong interactions between the DMAEH + and H 2 O trigger the formation of an orientated hydrogen-bonded network that could help to stabilize the lamellar structure and connect the successive layers separated by up to 90 nm. ( b ) The amount of intercalated DMAE molecules (as a percentage of the exchange capacity) provided as a function of the initial DMAE concentration. The amount of intercalated DMAE molecules first increased sharply in a nearly linear manner until reaching a saturation value at DMAE/H + = ~0.5–1, which is ~37% of the exchange capacity. This corresponded with the maximum swelling, beyond which no additional solvent could penetrate between the sheets. ( c ) A comparison of the DMAE concentrations inside and outside of the gallery. The DMAE typically concentrates in the gallery. Under the dilute regime before saturation, the external concentrations approached zero, while the internal concentrations remained nearly constant (0.04 mol l −1 ). The reverse occurred at high concentrations, beyond which little change in swelling was observed. ( d ) The radial distribution functions g ( r ) of water from nitrogen in TBAOH and DMAE and from oxygen (–OH) in DMAE. The solid and broken lines denote the water oxygen and hydrogen, respectively. The water molecules surrounding DMAEH + exhibited substantially higher-ordered structures than the random state around the TBA + . Furthermore, the –NH and –OH in the DMAEH + attracted O and H, respectively, of the polar H 2 O, producing water clusters with a net dipole ( Supplementary Fig. S8 ). The ‘polar’ water clusters interconnected through the dipole–dipole interactions, which may have helped to stabilize the highly swollen structure. Full size image To explore the equilibrium conditions, we evaluated both the intercalated quantity ( Fig. 4b ) and concentration of the DMAE ( Fig. 4c ) in the two regions. The intercalated DMAE values were determined by subtracting the amount of equilibrated DMAE molecules in the supernatant from the initial quantity, each of which was determined by titration with certain HCl standard solutions. The quantity of water entering the gallery was obtained from the spatial volume between the layers. In the dilute regime, almost all DMAE molecules (above 90%) entered into the gallery, and the quantity of intercalated DMAE increased linearly with the DMAE dose before reaching saturation at DMAE/H + =~0.5–1, which is ~37% of the exchange capacity. The value is comparable to the critical uptake value, ((C 4 H 9 ) 4 N) 0.3 H 0.4 Ti 1.825 O 4 ·H 2 O [8] , for inducing the delamination of titanate by tetrabutylammonium (TBA) ion that is known to be among the most effective delaminating reagents for a variety of layered compounds. We believe that this is not a coincidence and that it could be the result of the relatively unselective nature of acid–base reactions, which initiate the swelling and serve as a major driving force for the molecular mobility. The volume of associated water influx, which is determined by the osmotic pressure equilibrium between the internal and external regions, was proportional to the quantity of intercalated DMAE, producing a nearly constant internal electrolyte concentration. The external concentrations approached zero. Even with substantial increases in the initial DMAE concentrations, the DMAE molecules were typically concentrated in the gallery of the swollen crystals because of the Gibbs–Donnan equilibrium. [23] The Gibbs–Donnan equilibrium describes the effect of the impermeable macro-ions on the distributions of permeable ions across a semipermeable membrane, causing the concentration of counterions in the solution that contains the impermeable species to remain elevated even at equilibrium. In this work, the presence of unmovable negatively charged host sheets caused the interlayer region to contain a higher concentration of cations (DMAEH + ) while remaining electrically neutral. However, the situation was reversed at high DMAE concentrations (DMAE/H + >10), above which little change in swelling was detected. The swelling produced in highly concentrated solutions (DMAE/H + =100) yielded the same spacing found in samples swollen at DMAE/H + =20, except that the reflections were sharper and stronger. Furthermore, rather than swelling homogeneously, the original H 0.8 [Ti 1.2 Fe 0.8 ]O 4 ·H 2 O microcrystals tended to aggregate upon the addition of such concentrated solutions. Surprisingly, the layers with a separation distance of up to 90 nm were primarily spaced apart by H 2 O because the DMAE saturation value, which was ~37% of the exchange capacity, suggested that little space was occupied by the DMAE; an average of one DMAE molecule on the angstrom scale was contained in a voluminous H 2 O column with base area of 3 titanate unit cells (0.342 nm 2 ) and a height of 90 nm. However, unlike the previously reported swollen crystals, such as in tetrabutylammonium hydroxide (TBAOH) solutions, [6] , [8] , [9] that tended to naturally cleave into thinner particles as the intersheet separation exceeded ~10 nm, the swollen phase in this study was unusually stable. Agitation via manual shaking caused little change in the swollen crystals, whereas such treatment produced fragmentation or exfoliation of the crystals in the TBAOH solutions. Even with severe mechanical shaking, exfoliation was not observed apart from minor fragmentation ( Supplementary Fig. S6 ). The layers were strongly held together, and a long-range positional and orientational order was maintained, although the successive layers were separated by up to ~90 nm, a distance at which van der Waals forces or electrostatic attractions are weakened. Therefore, one would expect that other ‘adhesive’ forces were at work in this case. Ions in highly polar solvents such as H 2 O can usually lead to an ordered arrangement of water dipoles around a solute molecule. [24] , [25] The stability of the water shell varies widely depending on the interactions between the ions and H 2 O molecules. A simple estimation of the forces between the ion and H 2 O was performed (see Supplementary Methods and Supplementary Fig. S7 ) and suggested much stronger interactions in the DMAE case. Thus, the water molecules around the DMAEH + may exhibit a higher tendency towards order and may form a directional hydrogen-bonded network. The difference between the water around DMAEH + and TBA + was further examined using first-principle calculations of the radial distribution functions of the hydrations ( Fig. 4d ; Supplementary Fig. S8 ). The results for TBA + demonstrated only random distributions around one, suggesting no formation of hydration shells (left graph in Fig. 4d ). Conversely, several defined peaks occurred in the DMAEH + case, showing a structuring of the water molecules up to 9 Å at least. The H 2 O molecules directed themselves differently towards the N (–NH(CH 3 ) 2 ) and O (–OH) of the DMAEH + . Although the oxygen on the water molecules was closer to the nitrogen site than the hydrogen in the first hydration shell, the hydrogen was more strongly attracted to the O (–OH) site (middle and right graphs in Fig. 4d ). These results suggest that the DMAEH + and its hydration shells formed a kind of nanoscale hydration cluster that possessed a certain dipole. The dipole–dipole interactions among these directional clusters could mediate the 90-nm-range interactions between the layers. Recalling the fact that the internal DMAE concentration before saturation or the minimum concentration was roughly constant at 0.04 mol l −1 ( Fig. 4c ), if we simplify the hydration shell to a spherical shape, the radius would be ~2.1 nm (see Supplementary Methods for details). We believe that the strong ‘adhesive’ forces between the DMAEH + and H 2 O molecules and the possible formation of a continuous and oriented hydrogen-bonded network may help to stabilize the lamellar structure. In conclusion, we have realized the first case of instantaneous, reversible and extensive crystalline swelling of inorganic layered crystals. Unlike previous reports in which the swelling was limited or the crystals were readily cleaved into thinner pieces with extensive swelling, our work takes the generally perceived swelling to an extreme and unusual stage in which the crystals exhibit unexpected monolithic extensive swelling (up to ~100-fold or 90 nm at the maximum) and shrinking. The extraordinarily large space in the gallery was primarily occupied by H 2 O molecules, with a trace amount of the DMAE. Unlike the random H 2 O in the previously reported swollen phases that could be easily exfoliated, the long-range structuring of the H 2 O molecules in the highly swollen structure was confirmed using first-principle calculations, resulting in polar directional hydration clusters that likely help to stabilize the structure. The findings demonstrate important implications for and chemical insight into the exfoliating process and could aid in future research on the layered structure, exfoliation and 2D crystals. Furthermore, because of the significant water content (up to 97% in weight), the hydrogel of the highly swollen material could be produced through some general preparation methods, such as in situ polymerization. The hydrogel produced by mixing clay with a small proportion of a certain dendritic binder was highly mouldable and able to preserve biologically active proteins for catalysis. [26] The fluidity of water in confined geometries has long been of widespread interest, [27] , [28] and the distance between the layers of the stable swollen material is wide enough to be comparable to or exceed that of liquid crystalline phases, rendering the material an ideal model for basic studies regarding confined water or aqueous colloids. We believe that the work described herein could open a new avenue for such fundamental studies and potential applications. Synthesis procedures Dark-brown parent single crystals of K 0.8 [Ti 1.2 Fe 0.8 ]O 4 were obtained through a flux-growth method. In a typical procedure, a 1.2:0.4:2.03:1.63 mole ratio of the reagents TiO 2 :Fe 2 O 3 :K 2 CO 3 :MoO 3 , respectively, was thoroughly mixed in a mortar, loaded into a Pt crucible and tightly sealed. The crucible was then placed in a furnace preheated to 900 °C and held at that temperature for 30 min for decarbonation. After quenching, the powder was ground and calcined at 1,200 °C for 20 h. The K 0.8 [Ti 1.2 Fe 0.8 ]O 4 crystals were separated from the K 2 MoO 4 flux by dissolving them in water and then filtering. The transparent appearance under the optical microscope ( Fig. 1a ) indicated a high-quality product. The parent K 0.8 [Ti 1.2 Fe 0.8 ]O 4 single crystals were protonated in 0.5 mol l −1 HCl at ambient temperature, with a solution-to-solid ratio of 100 cm 3 g −1 . The sample turned yellow immediately after mixing with the HCl solution, and the system was stirred for 48 h with one intermediate replacement of the solution with fresh acid at 24 h. The H 0.8 [Ti 1.2 Fe 0.8 ]O 4 ·H 2 O crystals were collected via filtration, washed several times with water and dried in air. The swollen H 0.8 [Ti 1.2 Fe 0.8 ]O 4 ·H 2 O crystals were produced by mixing 100 cm 3 of an aqueous DMAE solution with a known mass of H 0.8 [Ti 1.2 Fe 0.8 ]O 4 ·H 2 O crystals (0.2 g), which was then allowed to remain still for 2 days to achieve equilibrium. The DMAE concentration ranged from 0.00086 to 0.1702, mol l −1 , which corresponded with a 0.1- to 20-fold excess to the exchange capacity of H 0.8 [Ti 1.2 Fe 0.8 ]O 4 ·H 2 O. Calculations of the radial distribution functions We calculated the radial distribution functions of the H 2 O molecules from N and O via first-principle molecular dynamics sampling. We used cubic supercells with a lattice constant of 1.973 nm. The DMAEH + cation and 251 H 2 O molecules were stuffed into the supercell in the DMAE case, while the TBA + case involved a TBA + cation with 245 H 2 O molecules. To maintain the charge neutrality under the periodic boundary condition and to mimic the presence of charged sheets, a background homogeneous charge (–1 e ) was introduced. The Nosé-Hoover thermostat method was used for the NVT ensemble. We used a simulation temperature of 353 K, which is typically considered appropriate for room temperature water in experiments. The time step was set at ~0.0967, fs, with 500 a.u. used as the fictitious mass of an electron in the Car-Parrinello dynamics. The electronic states and atomic forces in the entire system were calculated based on density functional theory. A plane-wave basis set at the energy cutoff of 70 Ry with norm-conserving pseudopotentials, and a G point was used to describe the Kohn–Sham orbitals. The BLYP functional was used for the exchange–correlation energy. After a few picoseconds, the equilibrium trajectories of all atoms were obtained. The snapshots of the trajectories are provided in Supplementary Fig. S8a . The radial distribution functions of the water oxygen and hydrogen from N in TBA + , N in DMAEH + and O (–OH) in DMAEH + were then calculated. How to cite this article: Geng, F. et al. Unusually stable ~100-fold reversible and instantaneous swelling of inorganic layered materials. Nat. Commun. 4:1632 doi: 10.1038/ncomms2641 (2013).